Carbon monoxide inhibits inward rectifier potassium channels in cardiomyocytes Reperfusion-induced ventricular fibrillation (VF) severely threatens the lives of post-myocardial infarction patients. Carbon monoxide (CO)—produced by haem oxygenase in cardiomyocytes—has been reported to prevent VF through an unknown mechanism of action. Here, we report that CO prolongs action potential duration (APD) by inhibiting a subset of inward-rectifying potassium (Kir) channels. We show that CO blocks Kir2.2 and Kir2.3 but not Kir2.1 channels in both cardiomyocytes and HEK-293 cells transfected with Kir. CO directly inhibits Kir2.3 by interfering with its interaction with the second messenger phosphatidylinositol (4,5)-bisphosphate (PIP 2 ). As the inhibition of Kir2.2 and Kir2.3 by CO prolongs APD in myocytes, cardiac Kir2.2 and Kir2.3 are promising targets for the prevention of reperfusion-induced VF. The reperfusion of myocardium subjected to a transient period of ischaemia rapidly induces severe ventricular arrhythmias [1] . Most cases of sudden cardiac death may result from reperfusion-induced ventricular fibrillation (VF) [2] . Such arrhythmias occur under a number of pathological and clinical circumstances [3] , [4] , [5] , and as such have stimulated a great deal of interest in the development of pharmacological agents to control reperfusion-induced VF. Haem oxygenase (Hmox) is the rate-limiting enzyme responsible for the degradation of haem in the endoplasmic reticulum to generate equimolar amount of biliverdin, free iron and carbon monoxide (CO) [6] . Myocardial expression of Hmox1 is upregulated in a rat experimental myocardial infarction model [7] . In mice lacking Hmox1 undergoing ischaemic/reperfusion, all the hearts examined exhibited VF [8] . The mechanism of ischaemia/reperfusion-induced VF involves the downregulation of Hmox1 mRNA and a reduction in Hmox activity [9] , however, the mechanism by which CO may act to prevent this remains unknown. CO is a promising molecule with therapeutic potential in a number of disorders due to its cytoprotective and homoeostatic properties [10] , [11] , [12] . The majority of endogenous CO is produced in a reaction catalysed by the enzyme Hmoxs [6] . CO is a potent vasodilator [13] and offers cardiac protection in myocardial ischaemia-reperfusion injury [9] . Here we investigated the effect of CO on ion channels, which contribute to action potential (AP) and identified a new subfamily of ion-channel targets for CO. CO prolonged ventricle AP duration by inhibiting Kir channels CORM-2 (tricarbonyldichlororuthenium (II) dimer [Ru(CO 3 )Cl 2 ] 2 , CO-releasing molecule) at the concentration of 10 μM and 1 μM significantly prolonged mean APD 90 (action potential duration at 90% repolarization) of rat ventricular myocytes by 68.7±4.54% ( P <0.001, n =5) and 35.6±3.24% ( P <0.001, n =5), respectively ( Fig. 1a ). 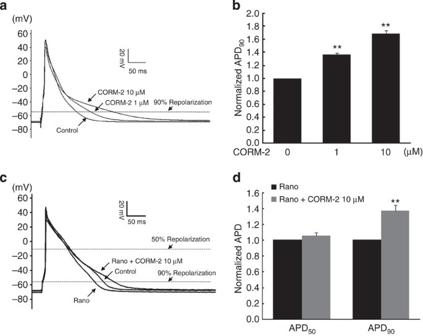Figure 1: CO prolonged APD of rat ventricular myocytes. (a,b) CORM-2 (10 μM and 1 μM) prolonged APD90of rat ventricles by 68.7±4.54% (n=5) and 35.6±3.24% (n=5), respectively. **P<0.001 versus control. (c,d) CORM-2 (10 μM) prolonged the APD50and APD90in the presence of 20 μM ranolazine (Rano) by 5.9±3.82% (n=6) and 37.0±7.38% (n=6), respectively. **P<0.001 versus Rano group. Figure 1: CO prolonged APD of rat ventricular myocytes. ( a , b ) CORM-2 (10 μM and 1 μM) prolonged APD 90 of rat ventricles by 68.7±4.54% ( n =5) and 35.6±3.24% ( n =5), respectively. ** P <0.001 versus control. ( c , d ) CORM-2 (10 μM) prolonged the APD 50 and APD 90 in the presence of 20 μM ranolazine (Rano) by 5.9±3.82% ( n =6) and 37.0±7.38% ( n =6), respectively. ** P <0.001 versus Rano group. Full size image CO chiefly extended the third period of repolarization. The possible candidate ion channels contribute to this prolonged AP include inward rectified K + currents (Kir2.0) and the sustained (late) component of the inward Na + current (late I Na ) (Na v 1.5) [14] . Ranolazine (Rano) is a common blocker for Na v 1.5 (ref. 15 ). It tonic blocks the late I Na with IC 50 of 5.6 μM, which are about 30–38-fold lower than required to cause tonic inhibition of peak I Na [15] , [16] , [17] . Application of ranolazine (20 μM) significantly reduced APD ( Fig. 1b ), suggesting the involvement of Na v 1.5 in the repolarization phase of AP. However, CORM-2 (10 μM) prolonged the APD in the presence of ranolazine (20 μM) by 37.0±7.38% ( P <0.001, n =6) ( Fig. 1b ), indicating that CO exerts its inhibitory effect partly through Kir2.0 channel. Additionally, the effect of ranolazine on CORM-2-induced prolongation of APD at the concentration of 80 μM was similar to its effect with 20 μM, suggesting that Rano at 20 μM was sufficient to completely block late I Na ( Supplementary Fig. 1 ). This is consistent to the previous report [14] . According to our results, the ratio, which represents the contribution of Na v 1.5 and Kir in the prolonged APs is approximately 3:4. To confirm whether CO could regulate the function of Kir2.0 channels, whole-cell patch-clamp was thereafter used to record the ionic currents of rat myocytes. The current–voltage (I–V) relationship of I Kir was recorded with ramp-like repolarizations in the presence and absence of CORM-2. The membrane was clamped to 0 mV for 50 ms and then repolarized from +40 to −140 mV at a rate of −100 mV s −1 repeated once every second. For I Kir recordings, Na + current was inactivated by holding at 0 mV and Ca 2+ current was inhibited by the addition of 10 mM nitrendipine to the bath. Strikingly, CORM-2 at the concentration of 10 μM markedly blocked I Kir by 34.43±4.27% at a holding potential of −120 mV ( P <0.001, n =5) ( Fig. 2a ). To further exclude other possible candidate ion channels in addition to Kir2.0 which is sensitive to Ba 2+ (1 mM), CORM-2 was applied in the presence of Ba 2+ . The fact that CO could not further extend the inhibition of Ba 2+ confirmed that CO-target ion channels are Ba 2+ -sensitive Kir2.0 ( Fig. 2b ). 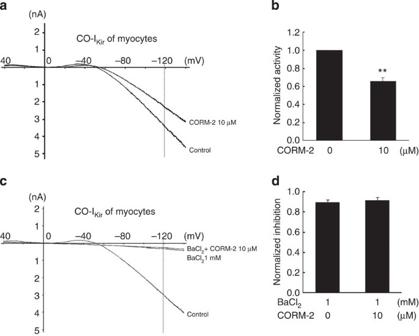Figure 2: CO inhibited rat myocardial IKir. (a,b) CORM-2 (10 μM) inhibited rat myocardial IKirby 34.43±4.27% at a holding potential of −120 mV (n=5).**P<0.001 versus control. (c,d) CORM-2 (10 μM) further inhibited IKirby 2.23±5.59% in the presence of Ba2+at a holding potential of −120 mV (n=5).P>0.05 between compared groups. Figure 2: CO inhibited rat myocardial I Kir . ( a , b ) CORM-2 (10 μM) inhibited rat myocardial I Kir by 34.43±4.27% at a holding potential of −120 mV ( n =5). ** P <0.001 versus control. ( c , d ) CORM-2 (10 μM) further inhibited I Kir by 2.23±5.59% in the presence of Ba 2+ at a holding potential of −120 mV ( n =5). P >0.05 between compared groups. Full size image CO blocked Kir2.2 and Kir2.3 but not Kir2.1 channels Human Kir2.2, Kir2.3 and Kir2.1 (KCNJ12, KCNJ4 and KCNJ2) which constitute human myocardial I Kir were individually expressed in HEK-293 cells to further clarify the effect of CO on Kir2.0. Barium chloride (BaCl 2 ), the specific inhibitor of Kir2.0 channels, was utilized to identify them. Results showed that CO remarkably inhibited the human Kir2.2 and Kir2.3 channels but not the Kir2.1 channel ( Fig. 3a–c ). The efficiency of CO on blocking Kir2.2 and Kir2.3 was determined by measuring the dose response of channel inhibition ( Fig. 3d ). Curve was plotted by the current size at −120 mV against the relative dosages and it was then fitted with non-linear Hill regression. The half-maximal inhibitory concentration (IC 50 ) of CORM-2 for Kir2.2 is 22.16 μM and the maximal inhibition was about 56.43±3.95% by 100 μM CORM-2. Meanwhile, the half-maximal inhibitory concentration (IC 50 ) of CORM-2 for Kir2.3 is 6.44 μM and the maximal inhibition was about 74.86±2.55% by 100 μM CORM-2. 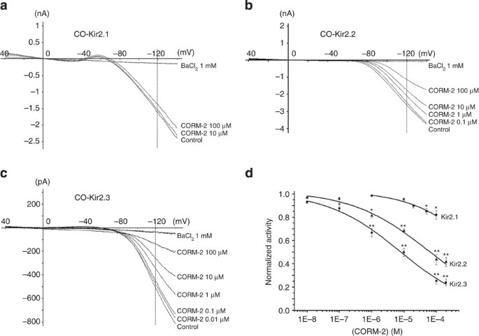Figure 3: CO specifically blocked Kir2.2 and Kir2.3 but not Kir2.1 channel expressed in HEK-293 cells. The inhibitory effect of CORM-2 at different concentrations on (a) Kir2.1, (b) Kir2.2 and (c) Kir2.3 currents. (d) Concentration-dependent inhibition by CORM-2 on Kir2.0 activity. Dosage curve was fitted with non-linear Hill. IC50=22.16, Hill coefficient is 0.992 (Kir2.2). IC50=6.44 μM, Hill coefficient is 0.995 (Kir2.3). **P<0.001, *P<0.01 versus control,n=5 each point. Figure 3: CO specifically blocked Kir2.2 and Kir2.3 but not Kir2.1 channel expressed in HEK-293 cells. The inhibitory effect of CORM-2 at different concentrations on ( a ) Kir2.1, ( b ) Kir2.2 and ( c ) Kir2.3 currents. ( d ) Concentration-dependent inhibition by CORM-2 on Kir2.0 activity. Dosage curve was fitted with non-linear Hill. IC 50 =22.16, Hill coefficient is 0.992 (Kir2.2). IC 50 =6.44 μM, Hill coefficient is 0.995 (Kir2.3). ** P <0.001, * P <0.01 versus control, n =5 each point. Full size image CO decreased the open probability of Kir2.3 channels To gain insight into the mechanism on how CO affecting the Kir2.3 channel, we tested the effect of CO on properties of single Kir2.3 channel expressed in HEK-293 cells. A single-channel current was recorded with a pipette voltage of 70 mV using the excised inside-out configuration and was then identified by its unitary conductance (13~14.2 pS) and pharmacological sensitivity. Application of 100 μM CORM-2 to the bath solution (intracellular side) inhibited the NPo of the Kir2.3 channel by 42.84±3.00% ( P <0.001, n =5) ( Fig. 4a ). No change of unitary conductance was observed. Common antagonists of Kir2.3 including BaCl 2 (1 mM) and genistein (100 μM) (a Kir2.3 channel-specific inhibitor [18] ) were also employed to compare the effect of CO on NPo of Kir2.3 ( Fig. 4b ). Our results showed a similar inhibitory effect on Kir2.3 for both CO and genistein. In addition, the time course of the CO inhibitory effect at a holding voltage of 70 mV was analysed ( Fig. 4c ). An example of long trace of single channels was shown as Supplementary Fig. 2 . CORM-2 at the concentration of 100 μM gradually decreased the NPo of Kir2.3 and this inhibition reached its maximum inhibition within 1 min. This inhibition outlasted the period of application and the NPo of Kir2.3 slowly recovered after washing out CO, suggesting a reversible and stable interaction between CO and the Kir2.3 channel. A similar inhibitory effect by genistein was observed. In contrast, BaCl 2 immediately decreased the NPo of Kir2.3 and exerted stronger inhibition. As membrane patches containing the channels are physically isolated from the rest of the cell in the inside-out configuration, cytoplasmic factors are largely absent. This indicates that CO directly inhibits the Kir2.3 channel current independent of the intracellular signal pathway. 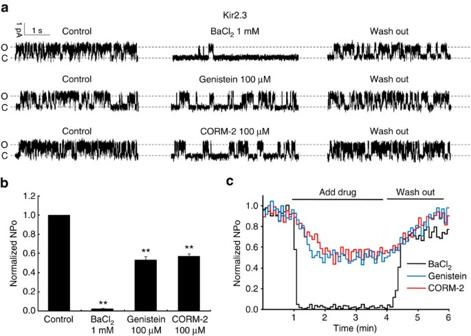Figure 4: CO directly decreased the open probability (NPo) of Kir2.3 channel. (a,b) The dotted lines labelled with ‘O’ and ‘C’ indicate the opened and closed state of Kir2.3 currents, respectively. (b) BaCl2(1 mM), genistein (100 μM) and CORM-2 (100 μM) decreased the NPo of Kir2.3 currents (at Vholding+70 mV) by 97.68±2.01%,n=4, 46.37±3.40%,n=5, 42.84±3.00%,n=5, respectively. After washing out the drugs, Kir2.3 current recovered entirely. **P<0.001 versus control. (c) Time course of CORM-2 (100 μM) action on Kir2.3 currents. Averaged NPo plot (5 s bins) from five repeated perfusions of indicated compounds were normalized to control. Figure 4: CO directly decreased the open probability (NPo) of Kir2.3 channel. ( a , b ) The dotted lines labelled with ‘O’ and ‘C’ indicate the opened and closed state of Kir2.3 currents, respectively. ( b ) BaCl 2 (1 mM), genistein (100 μM) and CORM-2 (100 μM) decreased the NPo of Kir2.3 currents (at V holding +70 mV) by 97.68±2.01%, n =4, 46.37±3.40%, n =5, 42.84±3.00%, n =5, respectively. After washing out the drugs, Kir2.3 current recovered entirely. ** P <0.001 versus control. ( c ) Time course of CORM-2 (100 μM) action on Kir2.3 currents. Averaged NPo plot (5 s bins) from five repeated perfusions of indicated compounds were normalized to control. Full size image CO regulated Kir2.3 by interfering its interaction with PIP2 A common feature of Kir2.0 channels is that they all require membrane phospholipid phosphatidylinositol (4,5)-bisphosphate (PIP 2 ) to maintain their activity [19] , [20] , [21] . The affinity of PIP 2 and Kir2.0 determines the sensitivity of Kir2.0 to many regulatory factors like pH, protein kinase C and membrane receptors such as type 1 muscarinic receptors (M1) and epidermal growth factor receptors [21] . Kir2.3 having a weak affinity with PIP 2 is sensitive to these regulators, whereas Kir2.1 possessing a strong affinity with PIP 2 is not sensitive to them. As described above, CO regulated Kir2.2 and Kir2.3 but not Kir2.1. We then asked whether the distinct effect of CO on Kir2.3 and Kir2.1 follows the same pattern and is partially due to PIP 2 . To test this hypothesis, we studied the effects of CO on Kir2.3 (T53I, I213L) and Kir2.1 (I79T, L222I) channel ( Fig. 5a,b ). Kir2.3 (T53I, I213L) is a mutant of Kir2.3 that has a stronger affinity with PIP 2 and behaves more like Kir2.1 regarding to its responses to inhibitory modulations [21] , [22] , [23] . Kir2.1 (I79T, L222I) is a mutant of Kir2.1, which has a weaker affinity with PIP 2 and behaves more like Kir2.3 (refs 22 , 24 ). The unitary conductance and NPo were not changed by mutation (data not shown). Results showed that CORM-2 at the concentration of 100 μM inhibited the NPo of Kir2.3 (T53I, I213L) channel by 12.29±2.79% ( n =5). The blocking effect was diminished significantly compared with wild-type Kir2.3 ( P <0.001, n =5), but was similar with that on Kir2.1. However, CORM-2 at the concentration of 100 μM significantly inhibited the NPo of the Kir2.1 (I79T, L222I) current by 39.64±3.28% ( P <0.001, n =5), which is similar with its effect on the Kir2.3 channel ( Fig. 5c ). 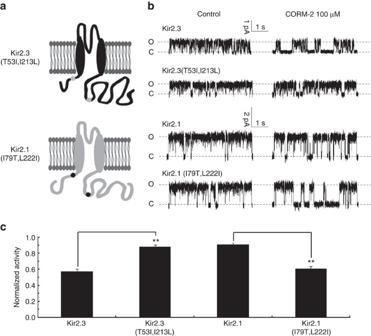Figure 5: CO regulated Kir2.3 channels by interfering the interaction between Kir2.3 channels and PIP2. (a) Mutant of Kir2.3 and Kir2.1 channels were constructed as shown in the left panel. (b,c) CORM-2 at the concentration of 100 μM inhibited Kir2.3 (T53I, I213L) currents by 12.29±2.79% (n=5). CORM-2 at the concentration of 100 μM remarkably inhibited Kir2.1 (I79T, L222I) by 39.64±3.28% (n=5). **P<0.001 compared with Kir2.3 and Kir2.1, respectively. Figure 5: CO regulated Kir2.3 channels by interfering the interaction between Kir2.3 channels and PIP 2 . ( a ) Mutant of Kir2.3 and Kir2.1 channels were constructed as shown in the left panel. ( b , c ) CORM-2 at the concentration of 100 μM inhibited Kir2.3 (T53I, I213L) currents by 12.29±2.79% ( n =5). CORM-2 at the concentration of 100 μM remarkably inhibited Kir2.1 (I79T, L222I) by 39.64±3.28% ( n =5). ** P <0.001 compared with Kir2.3 and Kir2.1, respectively. Full size image Additionally, CORM-2 was applied alone or in the presence of diC 8 -PIP 2 (the eight-carbon long acyl chains on PIP 2 , a synthetic water-soluble analogue of PIP 2 ) pre-loaded via the patching pipette. PIP 2 significantly rescued the inhibitory effect of CO on Kir2.3 expressed in HEK ( Fig. 6a,b ) and on I Kir currents in the ventricles ( Fig. 6c,d ). These results indicated that Kir2.3 was regulated by CO due to its low affinity with PIP 2 , implying that CO blocked Kir2.3 by interfering with the channel-PIP 2 interaction. 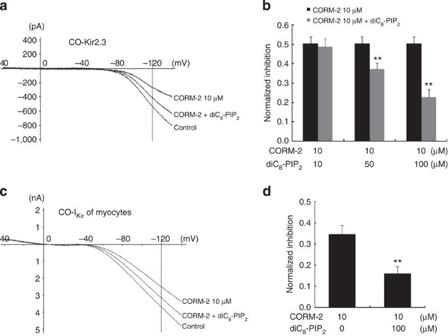Figure 6: DiC8-PIP2rescued the inhibitory effect of CO on myocardial IKircurrents. (a) Currents of Kir2.3 (expressed in HEK) in the presence of CORM-2 (10 μM) alone or with diC8-PIP2(100 μM). (b) CORM-2 (10 μM) alone inhibited Kir2.3 by 50.23±3.63%. In the presence of 10, 50 and 100 μM diC8-PIP2, CORM-2 (10 μM) inhibited Kir2.3 by 48.65±4.30%, 37.18±3.14% and 22.74±3.81%, respectively. **P<0.001,n=6 in each group. (c) Myocardial IKircurrents in the presence of CORM-2 (10 μM) alone or with diC8-PIP2(100 μM). (d) CORM-2 (10 μM) alone inhibited rat myocardial IKirby 34.44±4.28%. In the presence of 100 μM diC8-PIP2, CORM-2 (10 μM) inhibited rat myocardial IKirby 15.96±3.24%. **P<0.001,n=4. Figure 6: DiC 8 -PIP 2 rescued the inhibitory effect of CO on myocardial I Kir currents. ( a ) Currents of Kir2.3 (expressed in HEK) in the presence of CORM-2 (10 μM) alone or with diC 8 -PIP 2 (100 μM). ( b ) CORM-2 (10 μM) alone inhibited Kir2.3 by 50.23±3.63%. In the presence of 10, 50 and 100 μM diC 8 -PIP 2 , CORM-2 (10 μM) inhibited Kir2.3 by 48.65±4.30%, 37.18±3.14% and 22.74±3.81%, respectively. ** P <0.001, n =6 in each group. ( c ) Myocardial I Kir currents in the presence of CORM-2 (10 μM) alone or with diC 8 -PIP 2 (100 μM). ( d ) CORM-2 (10 μM) alone inhibited rat myocardial I Kir by 34.44±4.28%. In the presence of 100 μM diC 8 -PIP 2 , CORM-2 (10 μM) inhibited rat myocardial I Kir by 15.96±3.24%. ** P <0.001, n =4. Full size image In summary, we demonstrated that CO inhibited I Kir and prolongs APD in rat myocytes by regulating the interaction between Kir2.0 and PIP 2 , and profoundly inhibits Kir2.2 and Kir2.3 currents by decreasing the frequency of channel opening. According to the previous work [25] which studied the structural basis of PIP 2 activation of Kir2.2, the mutant Kir2.2 (I223L) (homologous to Kir2.3 (I213L) used in this study) affects conformation of the G-loop gate in a manner that might explain the apparent increased affinity for PIP 2 ; compared with the wild-type Kir2.2, the G-loop of Kir2.2 (I223L) adopts its PIP 2 binding conformation. Additionally, the rescuing effect of exogenous PIP 2 on CO inhibition ( Fig. 6 ) indicates the affinity change in PIP 2 binding with Kir2.0 channels is one of keys. Dominant PIP 2 binding with Kir2.3 by the increase of PIP 2 concentration reduced the CO interference, resulting in the rescue of CO inhibition on Kir2.3. Nonetheless, based on the results of the wild type as well as the mutants Kir2.1 and Kir2.3, CO most likely modulates the Kir2.0 channel activity by affecting the channels’ interaction with PIP 2 . Prolonged AP plays a key role in slowing down heart rate and lengthening the refractory period of myocytes. This may contribute to the prevention of reperfusion-induced VF. Very recent comprehensive analysis of regional ion-channel expression in normal and myopathic hearts documented that the ratio among Kir2.1, Kir2.2 and Kir2.3 is roughly around 13:7:8 in normal left ventricles and around 16:5:13 in myopathic left ventricles [26] . The elevation expression of Kir2.3 during the myopathic period pronounced the greater effect of CO in APD during the myopathy. It has been reported that Hmox1 was also significantly upregulated in myocardial infarction [7] , and its CO production was increased to protect the heart from reperfusion-induced VF [8] , [9] . Our results support this conclusion and underline the possible mechanism. Atrial fibrillation is a common arrhythmia and Kir2.3 is highly expressed in atrium [27] . As CO inhibits Kir2.3 current and prolongs APD in myocytes, it may cause slowing down of heart rates [28] , [29] , [30] and could be considered as a therapeutic target for AF. Kir2.0 has also previously been identified in mammalian forebrain [31] , [32] , [33] , nodes of Ranvier [34] , astrocytes [35] , heart [26] , [27] and renal epithelial cells [36] , serving important roles in setting membrane potential, modulating AP waveform and buffering extracellular K + . Increased Hmox1 expression has been found in Alzheimer’s disease brains [37] , [38] and its excessive product CO might cause depolarization and excitement of neuron by inhibition of Kir2.0. This new mechanism of the inhibitory effect of CO on Kir2.2 and Kir2.3 channels identifies a new physiological function of CO and offers a potential target for pharmacological and therapeutic application of CO by targeting Kir channels. Chemicals The methods in application of CO donor, tricarbonyldichlororuthenium (II) dimer [Ru(CO 3 )Cl 2 ] 2 (Sigma-Aldrich, St Louis, MO, USA) was freshly dissolved in DMSO as a stock solution. The medium containing a certain concentration of CO donor was made 30 min before experiments. The control group contains donor solutions which were placed at room temperature for 3 days to exhaust CO [39] . DiC 8 -PIP 2 was purchased from Echelon. Genistein was purchased from Sigma (Sigma-Aldrich, St. Louis, MO, USA). Ranolazine was purchased from Tokyo Chemical Industry. Animal experiments Animal experiments was approved by the Ethics Review Board for Animal Studies of IMM, Peking University. Myocytes were prepared from ventricles by standard collagenase dissociation technique [40] . cDNA constructs Human Kir2.1 cDNA was cloned in human umbilical vein endothelial Cells. Kir2.1 (I79T, L222I) mutations were produced by Pfu mutagenesis with QuikChange kit (Stratagene, La Jolla, CA, USA). Human Kir2.2 cDNA was cloned in human ventricular myocytes. Human Kir2.3 and Kir2.3 (T53I, I213L) cDNAs were generously provided by Dr Hailin Zhang. All of the cDNAs above were confirmed with DNA sequencing (Majorbio, Shanghai, China). Patch clamping Conventional whole-cell and inside-out configurations of the patch-clamp technique were used in the electrophysiological study. Signals were amplified using an Axopatch 200B amplifier (Axon Instruments) and filtered at 1 kHz. Data acquisition and analysis were carried out using pClamp 9.0 (Axon Instruments) software. Patch electrodes were pulled from a horizontal micropipette puller ( P -1000, Sutter Instruments) and fire polished to final tip resistance of 4–6 MΩ when filled with internal solutions. For whole-cell recording on myocytes, the pipette solution contained (in mM): 100 potassium aspartate (Sigma-Aldrich), 30 KCl, 1 MgCl 2 , 5 HEPES, 5 EGTA, 4 K 2 -ATP, pH 7.3 (adjusted with KOH); the bath solution contained (in mM): 140 NaCl, 5.4 KCl, 1.8 CaCl 2 , 1 MgCl 2 , 5 HEPES, 10 glucose, pH 7.4 (adjusted with NaOH). For whole-cell recording on HEK-293 cells, the pipette solution contained (in mM): 140 KCl, 2 MgCl 2 , 10 HEPES, 0.1 EGTA, 4 K 2 -ATP, pH 7.3 (adjusted with KOH); the bath solution contained (in mM): 120 NaCl, 5 KCl, 1.5 CaCl 2 , 1 MgCl 2 , 10 HEPES, 10 glucose, pH 7.4 (adjusted with NaOH). For single-channel recording, the pipette solution (extracellular) contained (in mM): 145 KCl, 10 HEPES, 10 glucose, pH 7.4 (adjusted with KOH); the bath solution (intracellular) contained (in mM): 145 KCl, 1.2 MgCl 2 , 10 HEPES, 0.1 EGTA, pH 7.38 (adjusted with KOH). Single-channel activity was recorded at a pipette voltage of 70 mV. The data were acquired at 20 KHz and low-pass filtered at 5 kHz. During post-analysis, data were further filtered at 200 Hz. Single-channel events were listed and analysed by pclampfit 9.0 (single-channel search-in-analyse function). NPo, the product of the number of channels and the open probability, was used to measure the channel activity within a patch. In total, 50% threshold cross-method was used to determine valid channel openings. Initial (1-2 min) single-channel records were normally used as the control. The activity of Kir2.0 during application of chemicals was normalized to activity during the control period to assess the effects of chemicals on Kir2.0 activity. Statistics Data were given as the mean±s.e.m., ‘ n ’ is the number of cells studied. Paired t -test was used to compare channel activity before (control) and after the application of drugs. Effects of different treatments were assessed by normalizing activity (to pretreatment levels) and comparing groups by using one-way analysis of variance (SPSS 13.0, Cary, NC, USA). Dosage curve was fitted with non-linear Hill by using Originpro7.0 (OriginLab, Northampton, MA, USA). How to cite this article: Liang, S. et al . Carbon monoxide inhibits inward rectifier potassium channels in cardiomyocytes. Nat. Commun. 5:4676 doi: 10.1038/ncomms5676 (2014).